Plasticity of Hopx+type I alveolar cells to regenerate type II cells in the lung The plasticity of differentiated cells in adult tissues undergoing repair is an area of intense research. Pulmonary alveolar type II cells produce surfactant and function as progenitors in the adult, demonstrating both self-renewal and differentiation into gas exchanging type I cells. In vivo , type I cells are thought to be terminally differentiated and their ability to give rise to alternate lineages has not been reported. Here we show that Hopx becomes restricted to type I cells during development. However, unexpectedly, lineage-labelled Hopx + cells both proliferate and generate type II cells during adult alveolar regrowth following partial pneumonectomy. In clonal 3D culture, single Hopx + type I cells generate organoids composed of type I and type II cells, a process modulated by TGFβ signalling. These findings demonstrate unanticipated plasticity of type I cells and a bidirectional lineage relationship between distinct differentiated alveolar epithelial cell types in vivo and in single-cell culture. In the adult lung, millions of air-exchanging units, termed alveoli, facilitate the transfer of oxygen from inhaled air into the blood stream. Mature alveoli are composed of two major distinct epithelial cell types, type I and type II cells. Type I cells are thin, have a large surface area and lie in close contact with capillaries to facilitate gas exchange; they express podoplanin (Pdpn) and Ager (advanced glycosylation end product-specific receptor). Type II cells are cuboidal and are defined by the production and secretion of surfactant proteins, including surfactant protein C (Sftpc), stored in specialized lamellar bodies. Studies in the 1960s and 1970s demonstrated that type II cells proliferate in response to injury and suggested that they gave rise to type I cells [1] , [2] . Recent genetic fate-mapping experiments extended these findings and showed that type II cells function as progenitors in the adult lung during homeostatic conditions and upon type II cell ablation [3] , [4] . Lineage-labelled type II cells both self-renew and generate type I cells in vivo and in clonal three-dimensional (3D) organoid cultures ex vivo [3] , [4] . Elucidating the mechanisms by which alveolar cell types are maintained and regenerated after injury has important implications for normal respiratory physiology and disease, and for designing regenerative therapies. An important outstanding question, however, is whether type I cells can change their phenotype and participate in regenerative responses in vivo . An emerging paradigm in stem cell biology is that some tissues use ‘facultative’ progenitors that differentiate in one direction under physiological conditions but may de-differentiate or transdifferentiate during repair following injury [5] , [6] , [7] . Multiple studies have highlighted this phenomenon in invertebrates [8] , but few examples have been documented in mammals, especially involving post-mitotic differentiated cells [5] . Previous studies suggested that isolated type I-like cells can be induced to express non-type I cell markers in vitro [9] , [10] . However, it remains an open question as to whether and under what conditions type I cells exhibit a phenotypic switch in vivo . Here we demonstrate that adult, differentiated type I cells, marked by expression of the atypical homeodomain-containing protein Hopx, can, under repair conditions, both self-renew and give rise to type II cells. Under the same conditions, the differentiation of type II to type I cells increases. These findings reveal a bidirectional lineage relationship between the differentiated cell types of the alveolar epithelium in response to physiological need. Hopx marks bipotent embryonic alveolar progenitors Early lung development is characterized by branching morphogenesis that results in a bronchiolar tree [11] , [12] . Lineage-tracing studies have shown that early tip cells that express Id2 and Sox9 are multipotent, but evidence suggests that as development proceeds they become restricted in developmental potential and later give rise only to alveolar cell types [4] , [13] , [14] , [15] , [16] . However, the identity and in vivo potential of individual late distal progenitor cells are still incompletely understood, requiring new lineage markers. Hopx is first expressed in the embryonic lung at embryonic day (E) 15.5, as judged by immunohistochemistry for both native protein and a ‘knock-in’ reporter allele in which GFP and Flag are expressed in Hopx + cells [17] . Specifically, Hopx is robustly expressed in the stalk cells of terminal end buds and excluded from surrounding mesenchyme ( Fig. 1a ). Hopx is also detected in a subset of Sox9 + cells near the distal tips ( Fig. 1b ). A subset of these distal Hopx + cells also coexpress Sftpc, Pdpn and Ager ( Fig. 1a,c,d and Supplementary Fig. 1a,b ). Our previous studies have implicated Hopx as an important regulator of lung development [18] . Gene ontology analysis of microarray data from whole Hopx −/− and Hopx +/+ E16.5 lungs confirmed significant changes in the expression of genes categorized as relevant to regulation of lung development and glyco- and lipoprotein expression ( Supplementary Data Set 1 ). 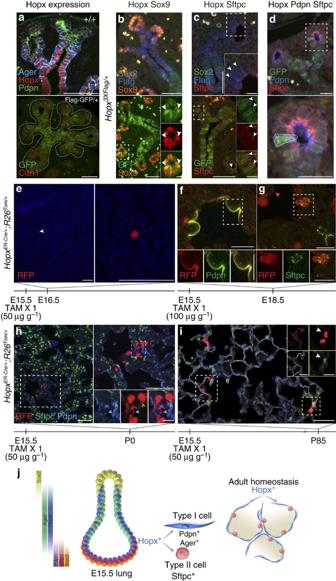Figure 1:Hopxmarks bipotent embryonic alveolar progenitors. (a–d) Sections of E15.5 lungs showing Hopx expression (Hopx3XFlag/+unless otherwise noted). (a) Hopx is expressed in distal epithelial cells and the stalk of developing alveolar buds. The top panel is stained with a Hopx antibody. (b) A subset of Hopx+cells coexpress Sox9. (Insets show boxed area and arrowheads point to Hopx+Sox9+cells.) (c) A subset of Hopx+cells coexpress Sftpc (insets show high magnification of boxed areas). (d) Rare Hopx+cells coexpress Pdpn and Sftpc (bottom panel is high magnification of boxed area in top panel with a triple-positive cell outlined). (e–i)HopxERCre/+; R26Tom/+embryos were exposed to one dose of tamoxifen at E15.5 and euthanized at indicated times. White arrowhead inepoints to single RFP+cell (magnified image to right). Red arrowhead ingpoints to lineage-labelled type I cell body and nucleus. Green and blue arrowheads inhpoint to a Sftpc+RFP+and Pdpn+RFP+cell, respectively. (j) Schema of Hopx expression at E15.5 in the developing lung. Scale bars, 10 μm (insets:b,c,h;f,g), 25 μm (iinsets) and 50 μm (a–e,i). Figure 1: Hopx marks bipotent embryonic alveolar progenitors. ( a – d ) Sections of E15.5 lungs showing Hopx expression ( Hopx 3XFlag/+ unless otherwise noted). ( a ) Hopx is expressed in distal epithelial cells and the stalk of developing alveolar buds. The top panel is stained with a Hopx antibody. ( b ) A subset of Hopx + cells coexpress Sox9. (Insets show boxed area and arrowheads point to Hopx + Sox9 + cells.) ( c ) A subset of Hopx + cells coexpress Sftpc (insets show high magnification of boxed areas). ( d ) Rare Hopx + cells coexpress Pdpn and Sftpc (bottom panel is high magnification of boxed area in top panel with a triple-positive cell outlined). ( e – i ) Hopx ERCre/+ ; R26 Tom/+ embryos were exposed to one dose of tamoxifen at E15.5 and euthanized at indicated times. White arrowhead in e points to single RFP + cell (magnified image to right). Red arrowhead in g points to lineage-labelled type I cell body and nucleus. Green and blue arrowheads in h point to a Sftpc + RFP + and Pdpn + RFP + cell, respectively. ( j ) Schema of Hopx expression at E15.5 in the developing lung. Scale bars, 10 μm (insets: b , c , h ; f , g ), 25 μm ( i insets) and 50 μm ( a – e , i ). Full size image To determine the fate of embryonic Hopx + cells, we performed lineage-tracing experiments using Hopx ERCre/+ mice and R26 reporter alleles [19] . To establish the validity of this approach, Hopx ERCre/+ ; R26 Tomato/+ ( R26 Tom/+ ) embryos were treated with a single dose of tamoxifen at E15.5 and lungs collected 24 h later. Lineage labelling results in nuclear and cytoplasmic RFP/Tomato expression and analysis confirmed the presence of a few, scattered, single Tom + cells ( Fig. 1e ) specifically within the distal domain of Hopx expression ( Supplementary Fig. 1c–f ). Lungs were then analysed at E18.5. Tom + cells coexpress either Pdpn ( Fig. 1f ) or Sftpc ( Fig. 1g ). At P0, we detected clusters of lineage-labelled cells that were composed of both type I and type II cells ( Fig. 1h ). Longer chases, up to 3 months postnatally, confirmed that Hopx-derived type I and type II cells are long lived ( Supplementary Fig. 2a,b ), and can be found in clusters, suggesting proliferation of Hopx-derived cells. ( Fig. 1i and Supplementary Fig. 2c,d ). Some of these clusters contained lineage-labelled type I cells intermixed with type II cells in discrete areas ( Supplementary Fig. 2d ). Taken together, the results from these lineage-tracing experiments are consistent with recent single-cell RNA-seq studies, suggesting that Hopx expression marks a bipotent alveolar progenitor [4] , [14] . Alveoli continue to mature postnatally (reviewed in ref. 20 ). When Hopx ERCre/+ ; R26 Tom/+ mice were given a single dose of tamoxifen at P5 and analysed at P28, both lineage-labelled type I and type II cells were identified ( Supplementary Fig. 2e,f ). However, labelling of Hopx cells at P35 and analysis at P46 revealed only lineage-labelled Pdpn + type I cells ( Supplementary Fig. 2g ). No Tom + Sftpc + could be identified among thousands counted ( Supplementary Fig. 2h ; 0/2334 Sftpc + cells were Tom + , n =3 mice). This suggests that during the first month of postnatal life, Hopx + normally becomes restricted to cells with the phenotype of differentiated type I cells ( Fig. 1j ). Hopx + cells give rise to type II cells during lung regrowth Analysis of the adult lung confirms that Hopx, a transcription cofactor [21] , is robustly expressed in the nuclei of cells that are type I, Pdpn + and Ager + ( Fig. 2a,b , red arrowhead). However, no expression is detected in Sftpc + type II cells ( Fig. 2c,d , 0/2276 Sftpc + cells observed in 22 sections, n =4 mice spanning P35–P133). We also failed to detect Hopx expression in Sftpc + and Scgb1a1 + cells, also known as bronchiolar alveolar stem cells [22] , at the bronchiolar alveolar duct junction ( Fig. 2e,f ). We performed short-term lineage tracing of Sftpc + cells by pulsing Sftpc ERCre/+ ; R26 Tom/+ ; Hopx 3XFlag/+ adult mice with tamoxifen every 5 days for 15 days (four doses); mice were killed 3 days later. We did not detect any Hopx-expressing (GFP + ) cells derived from adult Sftpc + cells (Tom + ) under homeostatic conditions ( Fig. 2g , 0/1847 Tom + cells were GFP + ), consistent with our earlier report [3] . Finally, quantitative RT–PCR (qRT–PCR) analysis of fluorescence-activated cell sorting (FACS) lineage-labelled Sftpc + and non-lineage-labelled Pdpn + alveolar cells from Sftpc ERCre/+ ; R26 Tom/+ adult mice is consistent with our conclusion that Hopx becomes restricted to type I cells in the adult alveolus and is excluded from type II, Sftpc + cells ( Fig. 2h ). 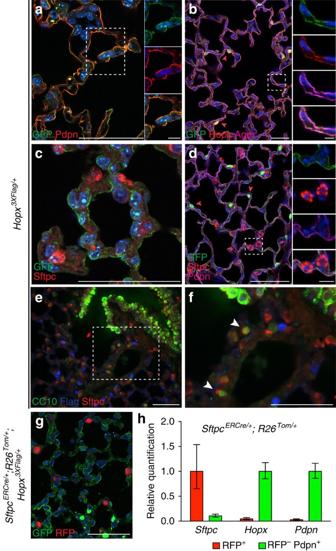Figure 2: Hopx is restricted to type I cells in the adult alveolus. (a–f) Hopx expression in the adult lung (Hopx3XFlag/+). Hopx is expressed in Pdpn+cells (a, P133) and Ager+cells (b, P38). Individual channels of boxed areas are shown as insets (a,b; merge is bottom inset in each panel). (c,d) Hopx is excluded from Sftpc+cells (c, P90d, P38). Red arrowheads highlight Hopx+, type I cell nuclei. (e,f) Sftpc+Scgb1a1+cells (arrowheads inf) do not express Hopx (boxed area inemagnified inf, P133). (g)SftpcERCre/+; R26Tom/+; Hopx3XFlag/+, P167 were dosed with tamoxifen every fifth day for 15 days total (four doses total) and euthanized at P186. GFP expression is distinct from Tomato expression. (h) As assayed by RT–PCR,HopxandPdpnare significantly enriched in the non-lineage-labelled, FACS-sorted type I cell population compared with the lineage-labelled, type II cell population. (Relative quantification (RQ) was normalized to 1 forHopxandPdpnin type I cell population; RQ 0.046 and 0.029 forHopxandPdpn, respectively in type II cell population.)Sftpcexpression is significantly lower in the type I cell population. (RQ normalized to 1 forSftpcin type II cell population; RQ 0.11 forSftpcin type I cell population.) Error bars:±95% confidence intervals. Scale bars, 10 μm (insetsa,b,d) and 50 μm (a–g). Figure 2: Hopx is restricted to type I cells in the adult alveolus. ( a – f ) Hopx expression in the adult lung ( Hopx 3XFlag/+ ). Hopx is expressed in Pdpn + cells ( a , P133) and Ager + cells ( b , P38). Individual channels of boxed areas are shown as insets ( a , b ; merge is bottom inset in each panel). ( c , d ) Hopx is excluded from Sftpc + cells ( c , P90 d , P38). Red arrowheads highlight Hopx + , type I cell nuclei. ( e , f ) Sftpc + Scgb1a1 + cells (arrowheads in f ) do not express Hopx (boxed area in e magnified in f , P133). ( g ) Sftpc ERCre/+ ; R26 Tom/+ ; Hopx 3XFlag/+ , P167 were dosed with tamoxifen every fifth day for 15 days total (four doses total) and euthanized at P186. GFP expression is distinct from Tomato expression. ( h ) As assayed by RT–PCR, Hopx and Pdpn are significantly enriched in the non-lineage-labelled, FACS-sorted type I cell population compared with the lineage-labelled, type II cell population. (Relative quantification (RQ) was normalized to 1 for Hopx and Pdpn in type I cell population; RQ 0.046 and 0.029 for Hopx and Pdpn , respectively in type II cell population.) Sftpc expression is significantly lower in the type I cell population. (RQ normalized to 1 for Sftpc in type II cell population; RQ 0.11 for Sftpc in type I cell population.) Error bars:±95% confidence intervals. Scale bars, 10 μm (insets a , b , d ) and 50 μm ( a – g ). Full size image In adult mice, unilateral pneumonectomy results in compensatory growth and ‘realveolarization’ of the remaining lung tissue [23] , including the formation of new secondary septa over a period of ∼ 2 weeks, but the source of new alveolar cells is not well defined (reviewed in ref. 24 ). To investigate whether type I cells contribute to the regrowth and remodelling, we gave a Hopx ERCre/+ ; R26 mt−mg/+ mouse a single dose of tamoxifen at P90 to lineage trace Hopx-expressing cells. Labelled cells expressed membrane-bound GFP. The left lung was then removed 19 days after tamoxifen administration ( Fig. 3a ). As expected, GFP + lineage-labelled Pdpn + type I cells were present in the alveoli of the resected lung segment ( Supplementary Fig. 3a ), and we could not detect any labelled Sftpc + cells that might have been derived from Hopx-expressing precursors ( Supplementary Fig. 3b ). The mouse was killed 7 days later and the remaining right-sided lobes were analysed. This revealed an increase in number of Hopx-derived, GFP + cells after pneumonectomy ( Fig. 3b–d ), many of which expressed Pdpn ( Supplementary Fig. 3c ). Consistent with this observation, there was an increase in the percentage of Hopx + that were phospho-histone H3 + at days 3 and 7 after pneumonectomy compared with sham, wild-type control mice ( Supplementary Table 1 ). At day 7, we also unexpectedly found rare Hopx-derived cells that expressed the type II marker Sftpc ( Fig. 3e–g ). We then repeated these experiments in Hopx ERCre/+ ; R26 Tom/+ mice using a single pulse of low-dose tamoxifen at P102 (50 mg kg −1 instead of 100 mg kg −1 , followed by a washout period averaging 20 days (range: 17–21 days, n =3) before pneumonectomy; Fig. 3a ). In these experiments, we analysed the remaining lungs 21 days after pneumonectomy and observed Hopx-derived Sftpc + cells that had persisted for at least this time ( Fig. 3h,i and Supplementary Fig. 4a–c ). Analysis revealed 18 Sftpc + , Hopx-derived cells out of a total of 656 Sftpc + cells counted ( ∼ 1 Sftpc + lineage-labelled cell per 700 μm 2 high-powered field in 16 sections, n =3 animals) compared with pre-pneumonectomy control samples in which 0/1156 Sftpc + cells were lineage labelled ( n =3 animals, at least three sections quantified from each; P <0.001, two-tailed t -test; Supplementary Fig. 4d ). These data indicate that by 21 days post pneumonectomy, ∼ 2.7% of type II cells are derived from Hopx + cells. However the Hopx ERCre/+ allele is relatively inefficient, with only 29±1.5% of Hopx + nuclei being lineage labelled at the time of pneumonectomy (average±s.d. ; Supplementary Fig. 4e ). This suggests that the contribution of type 1 to type II cells is in fact 9.4%. These experiments also confirmed an expansion of Hopx-derived alveolar cells (2.1-fold increase in percentage of Tom + nuclei post- versus pre-pneumonectomy, P =0.045, paired two-tail t -test; Supplementary Fig. 4f,g ), suggesting that Hopx + cells are capable of self-renewal. 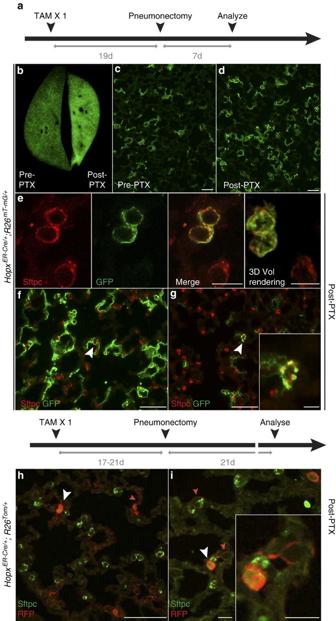Figure 3: Hopx+cells give rise to Sftpc+cells after pneumonectomy. (a) Schema of tamoxifen administration, pneumonectomy and euthanizing of mice. (b–f)HopxERCre/+; R26mT−mG/+mice were treated with tamoxifen at P90 and pneumonectomy or sham was performed at P109. Mice were euthanized 7 days later (b–g,n=1 mouse for each pneumonectomy and sham). Whole-mount immunofluorescence (b) and GFP expression in lungs pre- and post- pneumonectomy (c,d, respectively). (e–i) Post-pneumonectomy, Hopx-derived type I (red arrowhead) and type II (white arrowhead) cells were identified. Individual channels and merged image of a pair of adjacent Hopx-derived type II cells is shown ine, including a 3D volume rendering of a Z-stack through them (e, right panel). (f,g) Two more examples of Hopx-derived Sftpc+cells post pneumonectomy. (h,i)HopxERCre/+; R26Tom/+mice (n=3 each for sham and pneumonectomy) were pulsed with a single dose of tamoxifen (50 mg kg−1) at P102, pneumonectomy was performed at P118–P121 and mice were killed 21 days later. Insets ing,ishow high magnification of cell highlighted by white arrowhead. Scale bars, 10 μm (e,i;g,iinset) and 50 μm (c,d,f–h). Figure 3: Hopx + cells give rise to Sftpc + cells after pneumonectomy. ( a ) Schema of tamoxifen administration, pneumonectomy and euthanizing of mice. ( b – f ) Hopx ERCre/+ ; R26 mT−mG/+ mice were treated with tamoxifen at P90 and pneumonectomy or sham was performed at P109. Mice were euthanized 7 days later ( b – g , n =1 mouse for each pneumonectomy and sham). Whole-mount immunofluorescence ( b ) and GFP expression in lungs pre- and post- pneumonectomy ( c , d , respectively). ( e – i ) Post-pneumonectomy, Hopx-derived type I (red arrowhead) and type II (white arrowhead) cells were identified. Individual channels and merged image of a pair of adjacent Hopx-derived type II cells is shown in e , including a 3D volume rendering of a Z-stack through them ( e , right panel). ( f , g ) Two more examples of Hopx-derived Sftpc + cells post pneumonectomy. ( h , i ) Hopx ERCre/+ ; R26 Tom/+ mice ( n =3 each for sham and pneumonectomy) were pulsed with a single dose of tamoxifen (50 mg kg −1 ) at P102, pneumonectomy was performed at P118–P121 and mice were killed 21 days later. Insets in g , i show high magnification of cell highlighted by white arrowhead. Scale bars, 10 μm ( e , i ; g , i inset) and 50 μm ( c , d , f – h ). Full size image We performed two important control experiments to support the validity of our findings. First, sham-operated animals, in which the left lung was not removed, did not show any lineage-labelled Sftpc + cells 21 days after the operation ( Supplementary Fig. 5a–d , 0/1686 Sftpc + cells counted were Tom + , n =3 animals). Second, pneumonectomy of a Hopx 3XFlag/+ mouse at P102 did not result in any Hopx + and Sftpc + cells at 7 days (0/393 and 0/449 Sftpc + cells were Hopx + in sham-operated animals and post-pneumonectomy animals, respectively; Supplementary Fig. 5e–f ). This control shows that Hopx expression is not activated in Sftpc + type II cells in response to the regrowth stimulus. In parallel experiments, we performed pneumonectomies on Sftpc ERCre/+ ; R26 Tom/+ mice after treatment with tamoxifen to determine whether lineage-labelled type II cells give rise to type I cells during adult lung regrowth. Before pneumonectomy and in sham control animals, only DC-LAMP + cells in the alveoli were lineage-labelled cells (ref. 3 and Fig. 4a ), with little differentiation into type I cells, as previously described. DC-LAMP (Lamp3) is a glycoprotein found in lamellar bodies in mature type II cells. By contrast, 21 days post pneumonectomy, many lineage-labelled Hopx + type I cells were readily identifiable, particularly in the periphery of the lung ( Fig. 4b–d ; 16.0±5.2% RFP + cells were Hopx + , n =3 animals), where remodelling has been shown to be highest [24] . Taken together, our data show that during compensatory regrowth of the adult lung both Sftpc + type II and Hopx + type I cells contribute to the formation of new alveoli and undergo both proliferation and bidirectional differentiation. 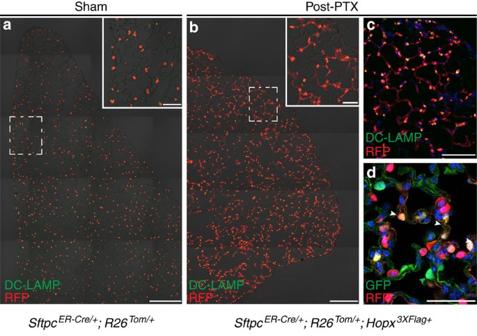Figure 4: Sftpc+cells give rise to type I cells after pneumonectomy. (a–d) Sham (a) or day 21 post-pneumonectomy (b–d) images fromSftpcERCre/+; R26Tom/+(a) andSftpcERCre/+; R26Tom/+;Hopx3XFlag/+mice (b–d). White arrowheads indpoint to lineage-labelled, GFP+type I cells. Green arrowhead indpoint to non-lineage-labelled Hopx+cells. DC-LAMP is a glycoprotein found in lamellar bodies in mature type II cells.n=3 mice for each sham and pneumonectomy experiments. Scale bars, 50 μm (a,binsets;d), 100 μm (c) and 200 μm (a,b). Figure 4: Sftpc + cells give rise to type I cells after pneumonectomy. ( a – d ) Sham ( a ) or day 21 post-pneumonectomy ( b – d ) images from Sftpc ERCre/+ ; R26 Tom/+ ( a ) and Sftpc ERCre/+ ; R26 Tom/+ ; Hopx 3XFlag/+ mice ( b – d ). White arrowheads in d point to lineage-labelled, GFP + type I cells. Green arrowhead in d point to non-lineage-labelled Hopx + cells. DC-LAMP is a glycoprotein found in lamellar bodies in mature type II cells. n =3 mice for each sham and pneumonectomy experiments. Scale bars, 50 μm ( a , b insets; d ), 100 μm ( c ) and 200 μm ( a , b ). Full size image Single type I cells form organoids ex vivo We sought to confirm our evidence for type I cell transdifferentiation using methods independent of Hopx ERCre/+ lineage tracing, and to further define the plasticity of individual Hopx + type I cells. We therefore adapted a 3D culture system for type II cells [3] to test the developmental potential of type I cells. In the original assay, individual type II cells both self-renew and give rise to type I cells, thereby forming 3D organoids. We hypothesized that individual Hopx + type I cells dissociated from these organoids would generate type II cell-containing organoids in clonal culture conditions. To test our hypothesis, adult Sftpc ERCre/+ ; Hopx 3XFlag/+ ; R26 Tom/+ mice were treated with tamoxifen, and 1–2 days after the final dose a single-cell suspension was prepared. Tom + (lineage-labelled type II) cells were isolated by FACS and plated at clonal density with Pdgfrα + stromal cells isolated from a separate cohort of mice ( Fig. 5a ). By day 16 of culture, organoids containing lineage-labelled Sftpc + type II cells and lineage-labelled (RFP + ) type I cells were present; the type I cells expressed GFP from the Hopx 3XFlag/+ allele ( Fig. 5b ). Spheres were then dissociated and lineage-labelled type II and type I cells were isolated, separated by FACS and replated individually in organoid culture. Within 14 days, both type I and type II cells gave rise to spheres ( Fig. 5c–h ). As previously described [3] , spheres derived from type II cells generated both type I and type II cells ( Fig. 5c–e ). Importantly, spheres derived from isolated type I cells were also composed of both type I and type II cells ( Fig. 5f–h ). We then dissociated type I-derived organoids ( Fig. 5f–h ), separated type I and type II cells based on differential endogenous Pdpn expression, and grew them again in organoid culture. Both cohorts of cells were able to generate organoids containing type I and type II cells, demonstrating that type I cells can give rise to Sftpc + , type II cells that retained the ability to self-renew and differentiate ( Supplementary Fig. 6a ). Therefore, we conclude that differentiated type I and type II cells can interconvert. 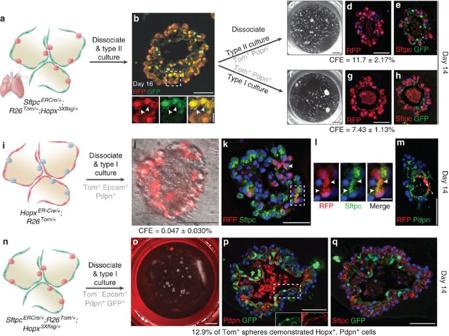Figure 5: Isolated Hopx+, type I cells give rise to type II cells in organoid culture. (a,b) Organoids grown fromSftpcERCre/+; Hopx3XFlag/+; R26Tom/+lineage-labelled type II cells (b) were dissociated and sorted into Type I (Tom+Pdpn+) and type II (Tom+Pdpn−) cells. Arrowheads inb(inset) point out RFP+Hopx+cell body. GFP only nuclei represent Pdgfrα+cells. (c–e) Type II-derived spheres. (f–h) Type I-derived organoids were composed of Sftpc+type II cells and Hopx/GFP+type I cells. (i–m) Organoids from type I cells (Epcam+Tom+Pdpn+) fromHopxERCre/+; R26Tom/+lineage-labelled alveoli. Rare mosaic spheres containing Tom+cells were observed on day 14. (k–m) Tom+cells coexpress Sftpc (k,l, arrowheads) and Pdpn (m). (l) High magnification of boxed area ink. (n–q) Organoids were generated from type I cells (Tom−Epcam+Pdpn+GFP+) fromSftpcERCre/+; Hopx3XFlag/+; R26Tom/+lineage-labelled alveoli. (o) Most spheres (mean=65 per well) were Tom−on day 14, and 12.9% of those were Hopx/GFP+. GFP−spheres likely derived from epithelial cells contaminating the stromal population. (p–q) Type I cell-derived organoid composed of Sftpc+type II cells and Pdpn+Hopx/GFP+type I cells. Note the cytoplasmic GFP expressed in Pdpn+cells, demonstrating that the organoid is not derived from the stromal population (insetp). Scale bars, 10 μm (binset;l), 50 μm (b,d,g,k,m,p,q), 100 μm (j) and 1,000 μm (c,f,o). Figure 5: Isolated Hopx + , type I cells give rise to type II cells in organoid culture. ( a , b ) Organoids grown from Sftpc ERCre/+ ; Hopx 3XFlag/+ ; R26 Tom/+ lineage-labelled type II cells ( b ) were dissociated and sorted into Type I (Tom + Pdpn + ) and type II (Tom + Pdpn − ) cells. Arrowheads in b (inset) point out RFP + Hopx + cell body. GFP only nuclei represent Pdgfrα + cells. ( c – e ) Type II-derived spheres. ( f – h ) Type I-derived organoids were composed of Sftpc + type II cells and Hopx/GFP + type I cells. ( i – m ) Organoids from type I cells (Epcam + Tom + Pdpn + ) from Hopx ERCre/+ ; R26 Tom/+ lineage-labelled alveoli. Rare mosaic spheres containing Tom + cells were observed on day 14. ( k – m ) Tom + cells coexpress Sftpc ( k , l , arrowheads) and Pdpn ( m ). ( l ) High magnification of boxed area in k . ( n – q ) Organoids were generated from type I cells (Tom − Epcam + Pdpn + GFP + ) from Sftpc ERCre/+ ; Hopx 3XFlag/+ ; R26 Tom/+ lineage-labelled alveoli. ( o ) Most spheres (mean=65 per well) were Tom − on day 14, and 12.9% of those were Hopx/GFP + . GFP − spheres likely derived from epithelial cells contaminating the stromal population. ( p – q ) Type I cell-derived organoid composed of Sftpc + type II cells and Pdpn + Hopx/GFP + type I cells. Note the cytoplasmic GFP expressed in Pdpn + cells, demonstrating that the organoid is not derived from the stromal population (inset p ). Scale bars, 10 μm ( b inset; l ), 50 μm ( b , d , g , k , m , p , q ), 100 μm ( j ) and 1,000 μm ( c , f , o ). Full size image We then confirmed that plasticity is a property of freshly isolated type I cells using two complementary approaches. Hopx ERCre/+ ; R26 Tom/+ mice were injected with tamoxifen to label type I cells, and 3 days later, type I cells were isolated by FACS (Tom + Epcam + Pdpn + ; Fig. 5i ). Isolated cells were placed in clonal organoid culture, and by day 14 lineage-labelled type I and type II cells were present ( Fig. 5j–m ). In a parallel approach, we cultured type I cells and lineage-labelled type II cells isolated by FACS from Sftpc ERCre/+ ; Hopx 3XFlag/+ ; R26 Tom/+ mice (Tom − Epcam + Pdpn + GFP + and Tom + Epcam + Pdpn − GFP − cells, respectively; Fig. 5n and Supplementary Fig. 6b ). qRT–PCR confirmed that Hopx and Sftpc were significantly enriched in the isolated type I and type II populations, respectively ( Supplementary Fig. 6c ). The type I cell-derived organoids were composed of Hopx/GFP + Pdpn + type I cells and Sftpc + type II cells ( Fig. 5o–q ). Taken together, the above experiments demonstrate that single Hopx + , type I cells possess the capacity to give rise to organoids composed of Pdpn + , type I cells, and Sftpc + , type II cells, ex vivo . In order to gain insight into the mechanism of type I cell to type II conversion, we repeated the organoid culture experiments as in Fig. 5a–h . We hypothesized that pathways known to be important regulators of lung development and homeostasis [24] , [25] , [26] , [27] , [28] also regulate the interconversion of type I and type II cells, and we used our organoid system to test the importance of candidate signalling pathways in this process. Specifically, organoids were prepared using lineage-labelled type II cells from Sftpc ERCre/+ ; Hopx 3XFlag/+ ; R26 Tom/+ mice. After 15 days in culture, organoids were dissociated into a single-cell suspension, and lineage-labelled type II and type I cells were isolated and separated by FACS. Triplicate samples of 3,000 cells of each phenotype were then replated at clonal density with Pdgfrα + fibroblasts in the presence of small molecules and agonists/antagonists of transforming growth factor-β (TGFβ), Wnt and Notch signalling pathways or vehicle control ( Fig. 6 ; and Supplementary Figs 7 and 8 ). 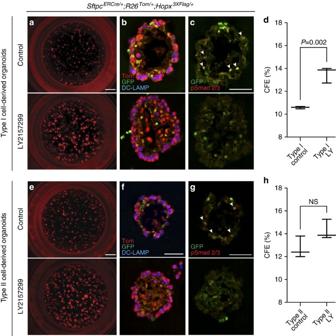Figure 6: Inhibition of TGFβ increases the rate of conversion of type I to type II cells in organoid culture. As inFig. 4, organoids grown fromSftpcERCre/+; Hopx3XFlag/+; R26Tom/+lineage-labelled type II cells were dissociated and separated into lineage-labelled type I cells (Tom+Pdpn+GFP+;a–d) and type II cells (Tom+Pdpn−GFP−;e–h). (a–d) Type I cell-derived organoids were grown in the presence of vehicle or the TGFβ inhibitor LY2157299 (LY). (b,c) Day 16 vehicle-treated organoids contain both type II cells (DC-LAMP+) and type I cells (HopxGFP+). Many GFP+type I cells are also pSMAD2/3+, suggesting active TGFβ signalling (white arrowheads). LY-treated organoids also contain both type II and type I cells, but they have reduced pSmad 2/3. (d) Day 14 CFE of LY-treated type I cells is significantly higher than vehicle control (n=3 replicates). (e–h) Type II cell organoids grown in the presence of LY also contain type II and type I cells (f), although there is no difference in the day 14 CFE between LY-treated organoids and control (h,n=3 replicates). Scale bars, 50 μm (b,c,f,g) and 1,000 μm (a,e). Figure 6: Inhibition of TGFβ increases the rate of conversion of type I to type II cells in organoid culture. As in Fig. 4 , organoids grown from Sftpc ERCre/+ ; Hopx 3XFlag/+ ; R26 Tom/+ lineage-labelled type II cells were dissociated and separated into lineage-labelled type I cells (Tom + Pdpn + GFP + ; a – d ) and type II cells (Tom + Pdpn − GFP − ; e – h ). ( a – d ) Type I cell-derived organoids were grown in the presence of vehicle or the TGFβ inhibitor LY2157299 (LY). ( b , c ) Day 16 vehicle-treated organoids contain both type II cells (DC-LAMP + ) and type I cells (HopxGFP + ). Many GFP + type I cells are also pSMAD2/3 + , suggesting active TGFβ signalling (white arrowheads). LY-treated organoids also contain both type II and type I cells, but they have reduced pSmad 2/3. ( d ) Day 14 CFE of LY-treated type I cells is significantly higher than vehicle control ( n =3 replicates). ( e – h ) Type II cell organoids grown in the presence of LY also contain type II and type I cells ( f ), although there is no difference in the day 14 CFE between LY-treated organoids and control ( h , n =3 replicates). Scale bars, 50 μm ( b , c , f , g ) and 1,000 μm ( a , e ). Full size image At 14 days of culture, we noted that treatment with 5 μM LY2157299 resulted in a significant increase in the colony-forming efficiency (CFE) of organoids derived from type I cells ( Fig. 6a–d ). CFE of organoids from type II cells was not significantly affected ( Fig. 6e–h ), but for both cell types the size of spheres was increased to about the same extent ( Fig. 6 and Supplementary Fig. 7 ). LY2157299 is a TGFβ receptor I kinase inhibitor that potently blocks the TGFβ signalling pathway by inhibiting the de-novo phosphorylation of pSmad2 (ref. 29 ). Consistent with a direct effect of the inhibitor on TGFβ signalling in epithelial cells, we identified Hopx + pSmad2/3 + cells in control spheres and a reduction in LY2157299-treated cultures ( Fig. 6c,g ). These data suggest that inhibition of TGFβ signalling preferentially augments the ability of a single type I cell to give rise to an organoid containing both type I and type II cells. Although pSmad2/3 was robustly expressed in Hopx + , type I cells in control cultures ( Fig. 6c,g ), we cannot rule out a non-cell autonomous effect of TGFβ inhibition in our culture system. Treatment of both type I and type II cultures resulted in larger organoids ( Supplementary Fig. 7 ). Treatment with recombinant TGFβ1 did not significantly affect CFE ( Supplementary Fig. 8a,b,f ), perhaps because the pathway is already stimulated under our organoid culture conditions. Modulation of the Wnt and Notch signalling pathways failed to augment type I to type II conversion ( Supplementary Fig. 8 ). Emerging reports suggest that adult stem and progenitor cell populations exploit a variety of mechanisms to maintain tissue homeostasis [5] , [8] , [30] , [31] . Previously, we demonstrated that the crypt of the mouse small intestine harbours two anatomically distinct populations of intestinal stem cells that are in dynamic equilibrium in steady state [19] . Our current findings with the adult lung suggest that interconversion can take place among differentiated cell types to maintain tissue integrity in the setting of repair in vivo . Prior work by our group and others [3] , [4] has demonstrated that adult type II alveolar cells can generate type I cells under homeostasis and partial type II cell ablation. Our present studies establish that the reverse is also true in vivo , and that a bidirectional lineage relationship exists between type I and type II cells during lung regrowth. Available tools and reagents do not allow us to determine whether conversion of type I cells to type II cells during regeneration necessitates ‘dedifferentiation’ to an embryonic-like bipotent state, or whether the conversion is ‘direct’. Regardless, it is clear that neither type I nor type II cells are ‘terminally’ differentiated and both retain unexpected plasticity into adulthood. These findings have important implications for regenerative medicine and for cancer. Indeed, interconversion of differentiated cell types makes discussion of the ‘cell of origin’ of certain cancers complex. Type II cells can be a cell of origin for lung adenocarcinoma based upon the analysis of tumours produced by activation of Kras in type II cells [4] , [32] , [33] . However, we found that Kras activation in Hopx + cells also produces tumours. Some tumours arising from Hopx + cells expressed Sftpc, suggesting that lineage plasticity may be hijacked during carcinogenesis ( Fig. 7 ). Ongoing studies focused on cellular reprogramming, and transdifferentiation coupled with increasingly sophisticated clonal analysis techniques may reveal unexpected plasticity in adult organs and tissues that contribute to homeostasis, tissue repair and disease. 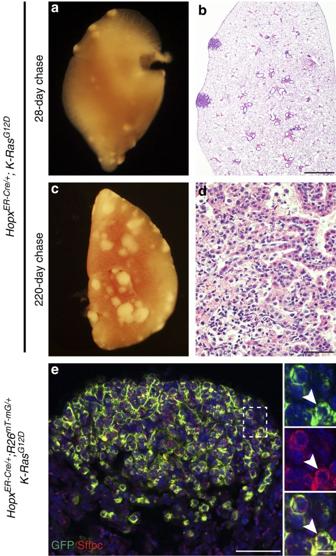Figure 7: Hopx+cells give rise to tumours in the lung. (a–e)HopxERCre/+; K-RasG12Dmice were pulsed with a single dose of tamoxifen between P90 and P100. (a,b) Within 28 days, peripheral tumours were formed. (c,d) Longer chases revealed tumours with aggressive features including atypical cells and high mitotic index (d). (e) Hopx-derived tumour cells (GFP+) inHopxERCre/+; R26mT−mG/+; K-RasG12Dexpress Sftpc. Individual channels of highlighted area are shown as insets. Arrowhead indicates aHopx-derived cell that is also Sftpc+. The mouse was pulsed with tamoxifen at P100 and killed 175 days later. Scale bars, 10 μm (einset), 50 μm (d,e) and 1,000 μm. Figure 7: Hopx + cells give rise to tumours in the lung. ( a – e ) Hopx ERCre/+ ; K-Ras G12D mice were pulsed with a single dose of tamoxifen between P90 and P100. ( a , b ) Within 28 days, peripheral tumours were formed. ( c , d ) Longer chases revealed tumours with aggressive features including atypical cells and high mitotic index ( d ). ( e ) Hopx-derived tumour cells (GFP + ) in Hopx ERCre/+ ; R26 mT−mG/+ ; K-Ras G12D express Sftpc. Individual channels of highlighted area are shown as insets. Arrowhead indicates a Hopx -derived cell that is also Sftpc + . The mouse was pulsed with tamoxifen at P100 and killed 175 days later. Scale bars, 10 μm ( e inset), 50 μm ( d , e ) and 1,000 μm. Full size image Hopx ERCre/+ , Hopx 3XFlag/+ , Sftpc ERCre/+ , K-Ras G12D/+ , R26 mT−mG/+ , R26 Tom/+ , Hopx LacZ/+ and B6.129S4- Pdgfra tm11(EGFP)Sor /J ( Pdgfra-H2B:GFP obtained from the Jackson Laboratory) mice have been described previously [3] , [17] , [19] , [21] , [33] , [34] , [35] . Hopx expression in the Hopx 3XFlag/+ allele can be detected by GFP or Flag expression, as a 3XFlag-viral-2A-GFP sequence was engineered into the 3′ UTR of the Hopx locus to append the final coding exon. Our previous studies demonstrate that GFP and Flag expression faithfully recapitulate Hopx expression [17] . A second, different R26 Tom/+ mouse allele [36] was used specifically in crosses performed that included Sftpc ERCre/+ . All mice were maintained on mixed genetic backgrounds. The University of Pennsylvania and Duke University Institutional Animal Care and Use Committee approved all animal protocols. Lineage-tracing experiments Mice were injected intraperitoneally or gavaged with 100 mg kg −1 body weight tamoxifen (Sigma) dissolved in corn oil unless otherwise indicated, as either a single or multiple doses, as indicated. For experiments represented in Fig. 2h , mice were injected every other day with 200 mg kg −1 body weight tamoxifen starting at P188 for a total of four doses; mice were killed at P196. For experiments represented in Fig. 4n , mice were dosed with 200 mg kg body weight tamoxifen for a total of four doses. Age of mice at time of tamoxifen injection is as indicated in the text and figures. Pneumonectomy Mice were anaesthetized with a mixture of ketamine (100 mg kg −1 ), xylazine (2.5 mg kg −1 ) and acepromazine (2.5 mg kg −1 ). Mice were then placed in the supine position, an endotracheal tube was inserted and mice were ventilated using a volume-cycled rodent ventilator (MiniVent Type 845; tidal volume of 0.4 ml room air, respiratory rate of 110 breaths per minute). The thoracic cavity was exposed by incising the fifth left intercostal space. The left lung was gently lifted through the incision, and then a 5-0 silk suture was tied around the hilum. The hilum was transected distal to the tie using forceps and microdissecting scissors ( n =4 mice total). Sham-operated mice ( n =4 total) underwent the identical surgical procedure, including isolating the left hilum, but without the resection of left lung. Hopx ERCre/+ ; R26 mT−mG/+ mice were pulsed with a single dose of tamoxifen (intraperitoneal, 100 mg kg −1 ) at P90 and pneumonectomy (or sham, n =1 for each condition) was performed at P109. The mice were killed 7 days after the surgery. Hopx ERCre/+ ; R26 Tom/+ mice were pulsed with a single dose of tamoxifen (intraperitoneal, 50 mg kg −1 ) at P102, and pneumonectomy (or sham, n =3 for each pneumonectomy and sham) was performed at P118–P121 (average washout period 20 days, range: 17–21 days) and mice were killed 21 days later. Lungs were visualized on a Olympus MVX10 fluorescent dissecting microscope. Sftpc lineage-labelled mice (related to Fig. 4 ; 11 weeks of age at time of tamoxifen administration; 16 weeks of age at killed) and C57/Bl6 mice (related to Supplementary Table 1 ; 10 weeks of age at killing) underwent sham or pneumonectomy as indicated in a similar fashion as that outlined above. All pneumonectomy experiments were performed with male mice (70–121 days old). Nuclei were identified based on 4,6-diamidino-2-phenylindole positivity or based on cellular morphology. Quantification was performed manually and using ImageJ software. Lung dissociation and FACS Lung dissociation and cell sorting was done as described previously [3] . In brief, lungs were inflated with a protease solution (2–3 ml per mouse; collagenase type I (450 U ml −1 ; Gibco), elastase (4 U ml −1 ; Worthington Biochemical Corporation), dispase (5 U ml −1 ; BD Biosciences) and DNaseI (0.33 U ml −1 ) in DMEM/F12); ref. 36 ), cut into small pieces and then incubated at 37 °C with frequent agitation. The resulting suspension was filtered, washed, incubated at room temperature in red blood cell lysis buffer (eBioscience), washed again and resuspended in DMEM+2% BSA. When antibody staining was required, lung suspension was blocked in 1% FcX TruStain (no. 101320; Biolegend) in 2% fetal bovine serum, 2% BSA in 1 × PBS. Antibodies used were: rat, Epcam-BV711 (1:800, no. 563134; BD Horizon); hamster, podoplanin-PE/Cy7 (1:250, no. 127412; Biolegend). Sorting was performed on FACS Vantage SE, and data were analysed with FACS Diva (BD Biosciences). For experiments related to Fig. 2h , a single-cell suspension from the lungs of Sftpc ERCre/+ ; R26 Tom/+ was made and first cells Tomato + were isolated via FACS (Tom + being lineage-labelled type II cells and their immediate derivatives). Tom − cells were then sorted based upon Pdpn expression to isolate type I cells (Tom − and Pdpn + ). For experiments related to Fig. 5a–h , cells Tom + cells were first isolated via FACS and then grown in organoid culture ( Fig. 5b ). Organoids from Fig. 5b were dissociated, Tom + cells were isolated via FACS based on Pdpn expression (Tom + , Pdpn + =type I cells, Tom + , Pdpn − =type II cells) and then grown in organoid culture. For experiments related to Fig. 5i–m , Tom+, Epcam + and Pdpn + cells were defined as type I cells and plated in organoid culture. For experiments related to Fig. 5n–q , Tom − cells were first isolated via FACS and then subsequently sorted based on Hopx/GFP and Pdpn expression. Tom − , Hopx + and Pdpn + cells were plated in culture (Hopx + , Type I cells). Organoid culture Stromal cells were obtained via FACS from Pdgfr α -H2B:GFP mice based upon GFP expression. As the GFP expressed by the Pdgfrα + stromal cells express is purely nuclear, it has an appearance unlike the GFP driven by Hopx expression in Hopx 3xFlag/+ mice, which is nuclear and cytoplasmic. Epithelial cells were sorted based upon lineage label and/or cell surface marker expression to discern type II and type I cells from all others. FACS-sorted cells were resuspended in MTEC/Plus and mixed 1:1 with growth factor-reduced Matrigel (BD Biosciences) [3] . Epithelial cells (5 × 10 3 ; unless otherwise indicated) and stromal cells (5 × 10 5 ) were seeded in 90 μl MTEC/Plus:Matrigel in individual 24-well 0.4-μm Transwell inserts (Falcon). CFE and histology were assessed between days 14 and 16. For passaging experiments, spheres were dissociated from Matrigel with the addition of 60 μl dispase to the insert and subsequent incubation at 37 °C for 30 min. Pdgfr α -H2B:GFP mice were wild type at the Hopx and Sftpc loci. For experiments related to Fig. 5a–h , Sftpc ERCre/+ ; Hopx 3XFlag/+ ; R26 Tom/+ mice, age 129 days or older, were pulsed four times with tamoxifen and killed 1–2 days after the final dose. For experiments related to Fig. 5i–m , Hopx ERCre/+ ; R26 Tom/+ mice were injected every other day (between P96 and P102) with tamoxifen, and 3 days later type I cells were isolated by FACS. For experiments related to Fig. 5n–q , Sftpc ERCre/+ ; Hopx 3XFlag/+ ; R26 Tom/+ mice were at least P43 or older. For the screen of candidate signalling pathways, the following small molecules/recombinant proteins were used: LY2157299 (Selleck; 5 μM), TGFβ1 (R&D; 0.2 ng ml −1 ), DBZ (Millipore; 1 μM), CHIR99021 (Tocris; 3 μM), XAV939 (Tocris; 1 μM) or vehicle control. Histology Lungs were fixed in 2% paraformaldehyde, ethanol dehydrated, embedded in paraffin and sectioned in the coronal plane, unless otherwise noted. Antibodies used were: GFP (goat, Abcam, and rabbit, Molecular Probes, 1:100–1:200), RFP (recognizes tdTomato; rabbit, Rockland, 1:250, and mouse, Abcam, 1:50–1:250), Sftpc (rabbit, Millipore, 1:250–1:500), Pdpn (mouse, Developmental Studies Hybridoma Bank, 1:50–1:100), Sox9 (rabbit, Santa Cruz, 1:100), Sox2 (rabbit, Seven Hills Bioreagents, 1:1,500 and goat, Santa Cruz, 1:500), Flag (mouse, Sigma, 1:100–1:250), Cdh1 (rabbit, Cell Signaling, 1:100), Hopx (rabbit, Santa Cruz, 1:100), Ager (rat, R&D, 1:50), phospho-histone H3 (mouse and rabbit, Cell Signaling, 1:20), DC-LAMP/CD208 (rat, Dendritics, 1:250) and phospho-Smad 2/3 (rabbit, Cell Signaling, 1:250). For Sftpc and RFP double staining, sections were first incubated 1:250–1:500 anti-Sftpc for 2 days at 4 °C. After washing, sections were incubated in 1:250 Alexa Fluo 488 AffiniPure Fab Fragment Goat anti-rabbit IgG (Jackson ImmunoResearch) for 2 h at room temperature. Subsequently, sections were co-stained with 1:50–1:250 anti-RFP and then the secondary antibody (1:250 Alexa Fluo 568 Goat anti-rabbit IgG or ImmPRESS Anti-Rabbit IgG). Further specific details of antibodies and immunhistochemistry are available upon request and basic staining protocols can be viewed at: http://www.pennmedicine.org/heart/research-clinical-trials/core-facilities/histology-gene-expression/ . For 3D imaging of whole-mount lung lobes, tissue was cleared with Sca l eA2 reagent (4 M urea, 0.1% wt/vol Triton X-100, 10% wt/wt glycerol in water [37] ). After fixation in 4% PFA and washing in PBS, tissue was placed in Sca l eA2 and kept on a rocker for 1–2 weeks at 4 °C until maximal tissue clearing occurred. Multiphoton images were acquired on an Olympus FV1000 with 25 × /0.9 numerical aperture ScaleView immersion lens. All immunohistochemistry was visualized on a Nikon Eclipse 80i fluorescence microscope, except the confocal images, which were evaluated on a Leica TCS SP8 or Zeiss 710 inverted confocal microscope. FIJI software was used to generate 3D volume rendering of a Z-stack images related to Fig. 3e (3D viewer plugin). All images were analysed using Adobe Photoshop (version CS6), ImageJ (version 1.0) and/or FIJI (version 1.49b; sizing, brightness or contrast adjustments and so on). Brightness and contrast were adjusted linearly across the entire image for any particular image, including individual colour channels for merged images. Quantitative real-time PCR Gene expression levels were quantified by qRT–PCR on the StepOne Plus Real-Time PCR System (Applied Biosystems). RNA was isolated using a RNAqueous-Micro Kit (Ambion) from three biological replicates for each experimental group. cDNA was synthesized using an iScript cDNA Synthesis Kit (Bio-Rad; 34.5 ng RNA used as template for experiment reported in Fig. 2h ; 30 ng RNA used as template for experiment reported in Supplementary Fig. 6c .) Samples were run in triplicate, and 18 μl reactions were pipetted from a master mix with 2 μl sample cDNA, 20 μl 2 × iQ SYBR Green Supermix, 10 μl water and 8 μl primers (200 nM each). Threshold cycle values (Ct) for triplicate samples were averaged and normalized to Gapdh (ΔCt), and these values across samples were compared (ΔΔCt) to quantify relative expression. Primers are as follows: Gapdh: forward 5′-AGGTCGGTGTGAACGGATTTG-3′, reverse 5′-TGTAGACCATGTAGTTGAGGTCA-3′; Sftpc: forward 5′-CAAACGCCTTCTCATCGTGGTTGT-3′, reverse 5′-TTTCTGAGTTTCCGGTGCTCCGAT-3′; Pdpn: forward 5′-ACCGTGCCAGTGTTGTTCTG-3′, reverse 5′-AGCACCTGTGGTTGTTATTTTGT-3′; Hopx: forward 5′-TTCAACAAGGTCAACAAGCACCCG-3′, reverse 5′-CCAGGCGCTGCTTAAACCATTTCT-3′. Data are reported as relative quantification; error bars represent 95% confidence intervals. Microarray analysis Microarray analysis was performed using three independent samples of Hopx +/+ and Hopx LacZ/LacZ (null) lung tissue from E16.5 embryos. RNA was extracted and reverse transcribed without amplification. Microarray analysis was performed by the University of Pennsylvania Microarray Core Facility using Affymetrix mouse cDNA arrays (Affymetrix Mouse Genome Arrays 430 v2.0). CEL files were RMA normalized using Partek Genomics Suite v6.6, and SAM (Significant Analysis of Microarray) was used to analyse the data. Rma-normalized log2-transformed intensities are reported. The Supplementary Data Set includes information for genes with >1.2-fold or < −1.2-fold change in Hopx −/− tissues compared with control. Gene ontology analysis was performed with the top 1,500 genes that were upregulated based on fold change (since Hopx is known to be a repressor). Analysis was performed by inputting those Affymetrix Probe ID numbers into: http://david.abcc.ncifcrf.gov . Microarray data have been deposited in GEO under accession code GSE65755 . Statistical analysis Two-tailed t -test was used to analyse the percentage of lineage-labelled Sftpc + cells in each mouse from pneumonectomy experiments. Eighteen lineage-labelled Sfptc + cells were identified from 16 sections from three post-pneumonectomy animals. At least four sections were quantified from each animal. Paired two-tailed t -test was used to compare the percentage of RFP + cells pre- and 21 days post pneumonectomy. Three pre-pneumonectomy and three post-pneumonectomy replicates were compared, and at least three sections were quantified from each replicate. Two-tailed t -test was used to analyse the CFE and average sphere diameter of organoids. Two-tailed t -test was used to analyse the percentage of phospho-histone H3 + cells. Accession codes: Microarray data have been deposited in GEO under accession code GSE65755 . How to cite this article: Jain, R. et al . Plasticity of Hopx + Type I alveolar cells to regenerate Type II cells in the lung. Nat. Commun . 6:6727 doi: 10.1038/ncomms7727 (2015).